Magneto-tunable photocurrent in manganite-based heterojunctions Correlated electron oxide heterojunctions and their photovoltaic effect have attracted increasing attention from the viewpoints of both possible application to novel devices and basic science. In such junctions, correlated electron physics has to be taken into account in addition to conventional semiconductor modelling to explain distinctively emerging features. However, extracting novel functionalities has not been easy because it is not possible to predict their interfacial properties solely from their bulk characteristics. Here we describe a magneto-tunable photocurrent in a pn junction based on a correlated electron oxide La 0.7 Sr 0.3 MnO 3 combined with a semiconducting SrTiO 3 substrate. On applying an epitaxial strain, the photocurrent is enhanced threefold, which is increased 30% further by a magnetic field. Such a magneto-tunable effect is possible for only a narrow window of the correlated gap, which is itself adjusted by bandwidth and temperature. These results provide a guideline for utilization of correlated phenomena into the novel electronic devices. Heterojunctions composed of materials with dissimilar properties are at the core of contemporary device physics and have enabled useful functionalities through the interactions of electrons at the interface [1] , [2] , [3] , [4] , [5] , [6] , [7] . As canonical examples, we have perovskite oxide heterointerfaces, in which both the semiconductor (single-electron) physics and the correlated electron (many-body) physics interact and combine with each other to some extent. In LaAlO 3 /SrTiO 3 (STO), for example, both the correlated electron phenomena (such as interfacial superconductivity and ferromagnetism) and the semiconductor-like behaviour (such as band bending and accumulation of laterally conductive electrons) emerge at the interface between two wide-gap semiconductors [1] , [7] . In studies of such materials, most attention has been paid to the transport of majority carriers [8] , [9] , [10] , [11] , [12] , [13] , while the minority carrier dynamics have remained elusive, although these may be important for the application to electronic devices, such as solar cells and light-emitting devices. Recently, photovoltaic devices based on correlated electron oxides, such as multiferroics and correlated electron manganites, have been attracting increasing attention [3] , [4] . Furthermore, some interesting electronic processes, such as multiple carrier generation by a single photon, have been proposed in correlated electron solar cells. In these reports, correlated physics and conventional modelling based on semiconductor physics are well integrated [14] , [15] , [16] . The minority carriers, that is, electrons and holes, produced through this process can be separated by the built-in potential at the heterointerface and then collected as photocurrent [14] . It was found in some cases that the interfacial band profiles in such heterointerfaces can be well understood within the framework of a rigid-band scenario, and that the electron correlations play a minor role in determining the properties of these heterointerfaces [17] . In contrast, the electron correlation effect becomes dominant when the interfacial carrier density was modulated by external fields [18] . In this context, an investigation into the subtle balance and harmonization of the two physical scenarios is very important. Furthermore, the isotype heterojunction that is comprised of a correlated electron oxide and an STO semiconductor layer provides an excellent platform for such a study. Here, we address this issue by exploring the magneto-tunability of a pn junction based on a correlated electron oxide La 0.7 Sr 0.3 MnO 3 (LSMO). It is found that the photocurrent generated in the junction is enhanced by a factor of >3 by applying a crystallographic distortion to the LSMO. Simultaneous application of an external magnetic field of 6 T can further enhance the photocurrent by 30%. Our analysis reveals that the electron correlation in LSMO, tunable by an external field, has a considerable effect on the quasi-band profile of the heterointerface, and hence on the collection probability of minority carriers. Wide tunability of electron correlation in manganites enables us to find an optimum window of photocurrent enhancement and gives a clue as to the design of correlated electron solar cells. Crystal structure and electric transport of manganite films LSMO was chosen as it is a typical correlated oxide with a phase competition near the heterointerface [7] , [12] . First, we investigated the crystal structure and lateral transport properties of LSMO films grown on insulating STO substrates. Both (001)- and (110)-oriented STO substrates have been selected here. The LSMO ( a bulk ~3.876 Å) films were subject to an in-plane tensile strain from STO ( a ~3.905 Å) due to the lattice mismatch (approximately −0.74%) [19] . X-ray reciprocal space mapping was used to study the lattice structure of the LSMO films (see Supplementary Fig. 1 ). We found that the LSMO (001) film has tetragonal distortion ( Fig. 1a ), whereas the (110) film has monoclinic distortion ( Fig. 1b ) because of shear mode strain with a tilting structure along the [110] axis (90− α =0.5°), which is consistent with the reported results [20] , [21] , [22] , [23] . The tilting lattice of the (110) film shows a single domain across the whole sample. When the film thickness ( t ) is less than a critical value (~40 nm), the unit-cell volume of the LSMO films expands beyond the bulk value owing to the biaxial in-plain strain from the substrate. It was found that the expansion for the (110) film (0.98% with t =24 nm) is larger than that for the (001) film (0.89%) and this tendency becomes prominent near the interface [21] . 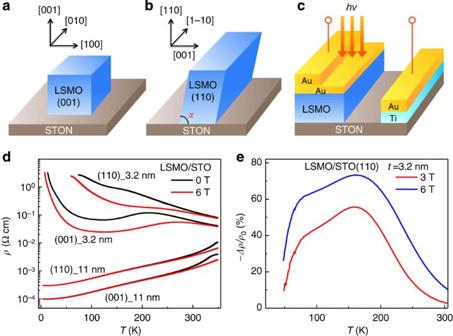Figure 1: Schematics of the samples and electrical transport properties of La0.7Sr0.3MnO3films. Crystal orientation and structure of (a) La0.7Sr0.3MnO3(LSMO) (001) and (b) LSMO (110) films on Nb-doped SrTiO3(STON) substrates. (c) Device structure for the photovoltaic effect measurements. (d) Temperature dependence of the resistivity for LSMO (001) and (110) films with different thicknesses deposited on Nb-free SrTiO3. The negative magnetoresistance is more pronounced for thinner films. (e) The relative change in resistivity (−Δρ/ρ0) as a function of temperature for the 3.2-nm-thick LSMO (110) film under 3- and 6-T fields. Figure 1d shows the resistivity for both the (001) and the (110) films with various thicknesses as functions of temperature and magnetic field. Comparing the (110) and (001) films at the same thickness, the tilt-distorted (110) films with larger cell-volume expansion exhibit higher resistivity than the (001) films, a trend more prominent in thinner films. For instance, the (110) film with t =3.2 nm shows a semiconductor-like transport behaviour even under a magnetic field of 6 T, while an insulator–metal transition is observed in the (001) film with the same thickness. The higher resistivity in (110) films may relate to the shear mode lattice strain or to the expansion of the cell volume [20] , [21] , but clarifying the detailed mechanism is beyond the scope of this work. On the whole, it is plausible to consider that the (001) interfaces are more conductive than those in the (110) case. The temperature dependence of magnetoresistance (−Δ ρ / ρ 0 ) for the 3.2-nm-thick (110) film is shown in Fig. 1e , indicating a peak around 175 K for both 3- and 6-T fields. Figure 1: Schematics of the samples and electrical transport properties of La 0.7 Sr 0.3 MnO 3 films. Crystal orientation and structure of ( a ) La 0.7 Sr 0.3 MnO 3 (LSMO) (001) and ( b ) LSMO (110) films on Nb-doped SrTiO 3 (STON) substrates. ( c ) Device structure for the photovoltaic effect measurements. ( d ) Temperature dependence of the resistivity for LSMO (001) and (110) films with different thicknesses deposited on Nb-free SrTiO 3 . The negative magnetoresistance is more pronounced for thinner films. ( e ) The relative change in resistivity (−Δ ρ / ρ 0 ) as a function of temperature for the 3.2-nm-thick LSMO (110) film under 3- and 6-T fields. Full size image Photovoltaic effect in manganite-based heterojunctions By combining an LSMO film ( t =24 nm) and an n -type Nb-doped (0.01wt%) SrTiO 3 (STON) substrate, rectifying heterojunctions were formed. The current density versus voltage ( J–V ) characteristics of the (001) and (110) junctions were measured with an illumination from a laser diode ( hv ~2.33 eV) under a magnetic field parallel to the film plane. The schematics of the junction device and experimental setup are shown in Fig. 1c . In dark conditions, both junctions have excellent rectification with J–V curves crossing the origin as shown in Fig. 2a,b . When the junctions are illuminated, the J–V curves are shifted downwards by the photocurrent. The illumination intensity was set at P =9.3 mW mm −2 which is a decade higher than a typical solar intensity (1 mW mm −2 ). The power density dependence of short circuit current ( J SC ) is shown as Supplementary Fig. 2 . Note the following two points from the comparison of Fig. 2a,b . First, the J SC for the (110) junction is larger than that of the (001) junction by a factor of three. Since the incident photon energy used here is lower than the band gap energy of STON ( E gs ~3.2 eV), only the excited photocarriers on the LSMO side contribute to the photocurrent. Therefore, the greater photocurrent in the (110) junction indicates a wider active interfacial layer than in the (001) junction [24] , [25] . Furthermore, the magnetic-field effect on the photocurrent is negligibly small in the (001) junction, while it is of significant magnitude in the (110) case. The J SC is enhanced by 12% through the application of 6 T at 150 K; this field-induced enhancement is almost linear with applied magnetic field, as shown in Fig. 2d . Moreover, the magnetic-field effect in the (110) junction is most prominent in the middle temperature range ( Fig. 2e ), and the relative change under 6 T, Δ J SC / J SC0 , has a peak around 150–200 K ( Fig. 2f ). This temperature dependence is similar to that observed in magnetoresistance ( Fig. 1e ). For the (001) junction, on the other hand, the magnetic-field effect is hardly observed across the entire temperature measurement range. As another reference, a junction composed of Pr 0.55 (Ca 0.7 Sr 0.3 ) 0.45 MnO 3 (PCSMO) and STON(110) has also been studied. Similar behaviour of photocurrent as (001) case were observed in PCSMO junction as shown in Fig. 2c . 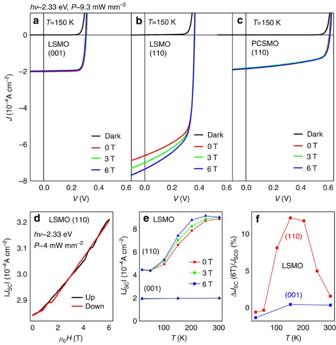Figure 2: Magneto-tunable photocurrent characterized by current density versus voltage measurements. (a–c) Current density versus voltage (J–V) relations for (001), (110) and PCSMO junctions, respectively. (d) Magnetic-field dependence ofJSCfor (110) junction with an illumination intensityP=4 mW mm−2. (e) Temperature dependence ofJSCfor both (001) and (110) junctions. (f) Temperature dependence of ΔJSC(μ0H=6 T)/JSC(0 T) for these junctions. Figure 2: Magneto-tunable photocurrent characterized by current density versus voltage measurements. ( a – c ) Current density versus voltage ( J–V ) relations for (001), (110) and PCSMO junctions, respectively. ( d ) Magnetic-field dependence of J SC for (110) junction with an illumination intensity P =4 mW mm −2 . ( e ) Temperature dependence of J SC for both (001) and (110) junctions. ( f ) Temperature dependence of Δ J SC ( μ 0 H =6 T)/ J SC (0 T) for these junctions. Full size image Electric transport of manganite-based heterojunctions To gain a deeper insight into the magneto-tunability in LSMO/STON junctions, the magnetic-field effect on the J–V characteristics and the junction capacitance ( C ) of (001), (110) and PCSMO junctions were investigated in dark conditions as shown in Fig. 3 . While all junctions show a highly rectifying diode property, the (110) junction has a relatively greater reverse saturation current density ( J S ) than does the (001) junction, which is consistent with previous results in La 0.6 Sr 0.4 MnO/STON junctions [26] . In addition, J S in the (110) junction can be modulated by the magnetic field, whereas there is no magnetic-field effect evident across the J–V range of the (001) junction. 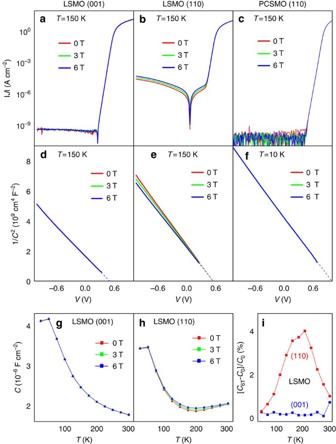Figure 3:J–Vand capacitance versus voltage characteristics obtained in dark condition. (a–c)J–Vcurves for (001), (110) and PCSMO junctions, respectively. (d–f) 1/C2–Vrelationships for (001), (110) and PCSMO junctions, respectively. The dashed lines are the results of linear fitting. (g,h) Temperature dependence ofCat zero bias for LSMO(001) and (110) junctions, respectively. (i) The temperature dependence of relative capacitance change [C6T−C0]/C0for LSMO(001) and (110) junctions. Figure 3d,e display the 1/ C 2 –V relationships of the (001) and (110) junctions, respectively. Fitting of 1/ C 2 –V curves with linear lines and their extrapolations onto the voltage axis (dashed lines) give the built-in potential ( V bi ) of the junctions, which are 0.50, 0.58 and 0.98 V for the (001), (110) and PCSMO junctions, respectively. Similar to the J–V relationships, the magnetic-field effect on C is negligibly small in the (001) junction across the bias voltage ( Fig. 3d ) and temperature ( Fig. 3g ) ranges, which is consistent with previous reports [17] , [26] . For the (110) junction, on the other hand, C is clearly enhanced by the magnetic field ( Fig. 3e,h ). We note that while the V bi of the (110) junction is not changed by the application of a magnetic field, the gradient of the 1/ C 2 –V curve decreases with increasing magnetic field. Again, this field-induced enhancement is temperature dependent, and the relative change [ C 6 T − C 0 ]/ C 0 has a peak around 150–200 K as shown in Fig. 3i . Figure 3: J–V and capacitance versus voltage characteristics obtained in dark condition. ( a – c ) J–V curves for (001), (110) and PCSMO junctions, respectively. ( d – f ) 1/ C 2 –V relationships for (001), (110) and PCSMO junctions, respectively. The dashed lines are the results of linear fitting. ( g , h ) Temperature dependence of C at zero bias for LSMO(001) and (110) junctions, respectively. ( i ) The temperature dependence of relative capacitance change [ C 6T − C 0 ]/ C 0 for LSMO(001) and (110) junctions. Full size image Although magnetic-field effects were observed in both J–V and C–V curves of the (110) junction, we consider their origins to be different. Numerical simulations have been performed for a semiconductor-based junction model taking shunt resistance ( R SH ) into account (for details, see Supplementary Fig. 3 ) [24] . The magnetic-field dependence of the J–V curve for the (110) junction in dark conditions can be well reproduced by changing R SH in simulation results. On the other hand, the same amount of change in R SH has negligible effect on C and photocurrent. These results indicate that the origin of greater J S in the (110) junction, and its change under magnetic fields, can be assigned to the shunt resistance, but the magnetic-field effects on J SC and C must originate from other factors. Photocurrent spectra of manganite-based heterojunctions The photocurrent density ( J ph ) is known to have a close relationship with the width of the depletion layers since J ph ~ qG ( W f +W s ), where G is the generation rate of photoexcited electron–hole pairs, W f and W s are the depletion-layer widths in LSMO and STON, respectively. In the constituent materials, the STON is magnetically inactive, while the magnetic field can modulate the electronic structure of LSMO, G and W f due to the strong correlation. The absence of the magnetic-field effect on J ph in the LSMO (001) junction indicates that W f is negligibly small or constant under magnetic fields. Considering that the interfacial layer in the LSMO (001) junction is rather metallic ( Fig. 1d ), W f will be negligible and thus we can regard it as a Schottky junction, shown schematically in the left inset of Fig. 4e , which is consistent with previous reports [13] , [17] . For the (110) junction with tilt-distorted LSMO film, in contrast, a more insulating interfacial layer ( Fig. 1d ) and magneto-tunable J ph and C signify the existence of a finite W f in the LSMO (110) side. Hence, the band profile of the (110) junction is rather close to the pn junction as schematically shown in the right two insets of Fig. 4e . 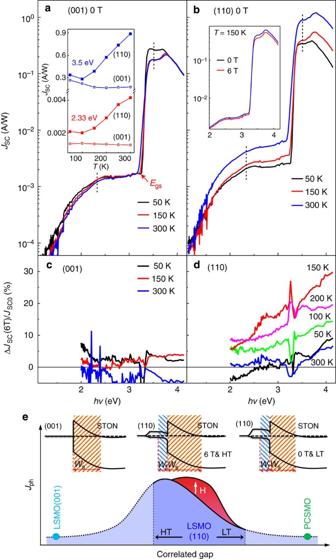Figure 4: Magnetic-field effect on photocurrent spectra of LSMO junctions. (a,b) Photocurrent spectra measured at various temperatures without magnetic field for (001) and (110) junctions, respectively. The inset inashows the temperature dependence ofJSCat selected photon energies of 2.33 and 3.5 eV (marked by dashed vertical lines inaandb). The upper inset inbshows photocurrent spectra under 0 and 6 T magnetic fields taken at 150 K. (c,d) Relative photocurrent change (ΔJSC/JSC0) with the application of a 6-T field as functions of photon energy and temperature for LSMO(001) and (110) junctions, respectively (Due to poor signal-to-noise ratio, data obtained belowhv=2 eV are omitted here). (e) A schematic image of the relationship betweenJSCand correlated gap in correlated junctions. The insets show the schematic band diagrams for (left) LSMO (001) junctions, (middle) LSMO (110) junction under high magnetic field (6 T) or high temperature (HT) and (right) LSMO (110) junction without magnetic field (0 T) or low temperature (LT), respectively. Figure 4: Magnetic-field effect on photocurrent spectra of LSMO junctions. ( a , b ) Photocurrent spectra measured at various temperatures without magnetic field for (001) and (110) junctions, respectively. The inset in a shows the temperature dependence of J SC at selected photon energies of 2.33 and 3.5 eV (marked by dashed vertical lines in a and b ). The upper inset in b shows photocurrent spectra under 0 and 6 T magnetic fields taken at 150 K. ( c , d ) Relative photocurrent change (Δ J SC / J SC0 ) with the application of a 6-T field as functions of photon energy and temperature for LSMO(001) and (110) junctions, respectively (Due to poor signal-to-noise ratio, data obtained below hv =2 eV are omitted here). ( e ) A schematic image of the relationship between J SC and correlated gap in correlated junctions. The insets show the schematic band diagrams for (left) LSMO (001) junctions, (middle) LSMO (110) junction under high magnetic field (6 T) or high temperature (HT) and (right) LSMO (110) junction without magnetic field (0 T) or low temperature (LT), respectively. Full size image The above scenarios on the interfacial band profiles and their magnetic-field effects are also supported by the photocurrent action spectra ( J SC versus hv ) as shown in Fig. 4 . For both (001) and (110) junctions, the J SC has a jump at around 3.2 eV (marked by an arrow in Fig. 4a ), which corresponds to the E gs of STON. The J SC above (below) E gs originates mainly from the photocarriers generated in the depletion layer of STON (LSMO). To draw further information on the depletion layer in each region, we plot the temperature dependence of J SC for photon energies below ( hv =2.33 eV) and above (3.5 eV) E gs in the inset of Fig. 4a . Below E gs , J SC is almost temperature independent in the (001) junction. Above E gs , J SC increases slowly at first with cooling and then increases rapidly at temperatures below 150 K. This feature reflects the variation of W s in STON ( W s ~ ε s 1/2 ), as is evident in the capacitance ( C j ~ ε s / W s ~ ε s 1/2 ) results shown in Fig. 3g . Moreover, it is found that the magnetic-field effect on J ph of the (001) junction is negligibly small across the whole spectrum ( Fig. 4c ) and is consistent with the J ph –V curves ( Fig. 2a ). As for the (110) pn junction with finite W f , the situation is quite different, where the temperature/magnetic-field-dependent correlated gap ( E gf ) plays an important role. In the correlated electron manganite, ‘Mottness’ is controlled by external fields [6] , [7] , that is, the temperature/magnetic-field dependence of the insulating gap in the LSMO interfacial layer is expected (the right two insets of Fig. 4e ). An increase in temperature or magnetic field brings out shrinkage of E gf and an enhancement of the effective carrier density ( n f ). As a result, on the one hand, the increase of n f can enhance on the STON side proportionally, while decreasing on the LSMO side [24] , n s being the carrier density of substrate and ε f the dielectric constant of the LSMO film. On the other hand, in accord with the shrinkage of E gf , the increase in temperature or magnetic field drives this correlated system closer to the phase boundary with metal. Then, the photocurrent, which is related to the phase stability, may be enhanced [14] , [15] . For the hv < E gs region, obviously, the latter factor is dominant, and higher temperature or higher magnetic field produces the larger J SC , as shown in Fig. 2e and the inset of Fig. 4a . For the hv > E gs region, the former factor, that is, W s on the STON side, is dominant for J SC . Then the enhancement of J SC can also be produced with an increase of temperature and magnetic field, as shown in Fig. 4b,d . The Δ J SC / J SC0 under 6 T ( Fig. 4d ) can reach up to ~30% with hv =4.1 eV at 150 K. These results indicate that the correlated gap E gf plays a decisive role in the magnitude of J ph and its temperature- and magneto-tunability in the correlated junction. This remarkable feature is summarized schematically in Fig. 4e . Zero E gf (for example, the (001) junction) with absence of W f results in a small J ph and negligible temperature and magnetic-field effects. The (110) junction with medium E gf can produce a greater J ph at high temperature or high magnetic field (left and up arrows in Fig. 4e ), and its value will be reduced again when the E gf increases further by lowering the temperature (right arrow) or removing the magnetic field. From this tendency, one can expect that a further increase of E gf , accompanying a robust insulating state against external fields, will result in smaller J ph as well as smaller temperature and magnetic-field effects. The results on the PCSMO junction with larger E gf verify this expectation ( Fig. 2c ). The PCSMO is in a highly robust insulating state at the interface and insensitive to small external magnetic fields used here. The most surprising and important finding in this study is that when the interface is in a phase-competing state (middle correlated gap) and the magneto-photocurrent effect is remarkable as in the LSMO (110) junction, the absolute magnitude of the photocurrent is simultaneously enhanced. This means that there is an optimum window of electron correlation for the effective harvest of photocurrent ( Fig. 4e ). One possible origin for the photocurrent enhancement we have in mind is the local phase transition from the gapped to metallic state near the interface. When the interface is in slightly gap-opened state and keen phase competition, it becomes most amenable to the photoexcitation. The present study reveals that the choices of the appropriate substrate orientation as well as the chemical composition are critical factors to tune the correlated gap and approach the optimum window. Sample preparation The LSMO films of 24 nm thickness were deposited on both (001) and (110) STON single-crystal substrates with 0.01wt% Nb-doping using a pulsed laser deposition technique. For the electrical measurements in the perpendicular direction, these junctions were patterned into a mesa-structure (400 × 600 μm 2 ) using a photolithographic technique. Light illuminated the junction through a semi-transparent Au electrode (5 nm thick). The details of the film growth and device fabrication have been reported elsewhere [17] . Electrical transport and magneto-photovoltaic measurements The J–V and C–V characteristics were measured with a semiconductor parameter analyzer (Agilent 4156C) and a precision LCR metre (Agilent E4980A), respectively. The measured frequency of C was 1 kHz. The photocurrent spectra were obtained by using lock-in detection, and the junctions were irradiated with a chopped monochromatic light produced by a monochromator (Acton SpectroPro. 2300i) and a halogen lamp. The J–V and C–V curves with photoirradiation were obtained with use of a continuous-wave laser. The laser power is below 25 mW and the radius of the beam spot is 920 μm. To reduce the heating effect, we put a shutter in front of the focusing lens, and the measurements were started just after opening the shutter (delay time is set as 200 ms) and it was closed soon after the measurements were completed. The illumination time for one measurement cycle is around 1 s. For all the electrical measurements, triaxial Bayonet Neill–Concelman cables were utilized in a magneto-optical cryostat equipped with a superconducting magnet (Oxford Instruments SM4000-8-M). How to cite this article: Sheng, Z. G. et al . Magneto-tunable photocurrent in manganite-based heterojunctions. Nat. Commun. 5:4584 doi: 10.1038/ncomms5584 (2014).